Atomic-scale insights on hydrogen trapping and exclusion at incoherent interfaces of nanoprecipitates in martensitic steels Hydrogen is well known to embrittle high-strength steels and impair their corrosion resistance. One of the most attractive methods to mitigate hydrogen embrittlement employs nanoprecipitates, which are widely used for strengthening, to trap and diffuse hydrogen from enriching at vulnerable locations within the materials. However, the atomic origin of hydrogen-trapping remains elusive, especially in incoherent nanoprecipitates. Here, by combining in-situ scanning Kelvin probe force microscopy and aberration-corrected transmission electron microscopy, we unveil distinct scenarios of hydrogen-precipitate interaction in a high-strength low-alloyed martensitic steel. It is found that not all incoherent interfaces are trapping hydrogen; some may even exclude hydrogen. Atomic-scale structural and chemical features of the very interfaces suggest that carbon/sulfur vacancies on the precipitate surface and tensile strain fields in the nearby matrix likely determine the hydrogen-trapping characteristics of the interface. These findings provide fundamental insights that may lead to a better coupling of precipitation-strengthening strategy with hydrogen-insensitive designs. The pledge of zero carbon dioxide emission has provoked an increasing demand on clean hydrogen to reduce the use of fossil fuels. However, hydrogen poses detrimental effects on the mechanical properties of metallic materials [1] , [2] , [3] , [4] , [5] , [6] , commonly known as hydrogen embrittlement (HE), which endangers the safe operation of structural materials such as high-strength alloys in energy-efficient vehicles [7] and hydrogen storage tanks [8] . Generally, hydrogen embrittlement sensitivity increases with the material strength, being a major concern in the development and practical application of high strength alloys. One of the most attractive methods to intervene and mitigate HE employs nanosized precipitates, which have demonstrated great efficacy in strengthening and toughening materials [9] , [10] , [11] , to trap and diffuse hydrogen atoms from enriching at vulnerable locations in the materials [12] , [13] , [14] . It is generally believed that hydrogen can be captured inside the alloy carbide nanoparticles and/or in proximity to their interfaces with the matrix, presumably by vacancies, specific interfacial structures, misfit strains, and/or threading dislocations [14] , [15] , [16] , [17] , [18] , [19] . Nevertheless, as for incoherent nanoprecipitates which may provide a deeper trap for hydrogen than the coherent and semi-coherent interfaces [20] , [21] , it remains contentious as for whether they can trap hydrogen. Thermal desorption spectroscopy (TDS) results indicate that incoherent precipitates such as TiC, NbC, and VC in steels do not trap hydrogen when the hydrogen is electrochemically charged into the material at room temperature [14] , [20] , [21] , [22] . On the contrary, atom probe tomography (APT) results solidly reveal deuterium segregation at the incoherent interfaces between the NbC and martensite matrix [23] . Depending on the precipitate/matrix mutual orientation, the structures of incoherent interfaces are intrinsically diverse and may presumably lead to different hydrogen-trapping behaviours. Therefore, ensemble-average methods such as the TDS are not sufficient to unravel the hydrogen-trapping characteristics of individual precipitates, not to mention the key underlying mechanisms. On the other hand, though APT can image the spatial distribution of hydrogen, it has to destruct the sample hindering further characterization on the trapping sites [24] . Here, by using a non-destructive method of scanning Kelvin probe force microscopy (SKPFM) for hydrogen detection, unprecedentedly, we in situ unveil the hydrogen trapping behaviours of individual incoherent nanoprecipitates within a high-strength low-alloyed steel. It is found that not all incoherent interfaces are trapping hydrogen introduced through electrochemical charging; some may even exclude hydrogen. Subsequent characterizations on the precipitates with aberration-corrected scanning transmission electron microscopy (STEM) unravel the structural and chemical origins of the diverse hydrogen trapping behaviours, identifying carbon/sulfur vacancies on the precipitate surface and tensile strain fields in the nearby matrix as key factors that capture hydrogen on the precipitate/matrix interfaces (simply referred to as interface in the following). 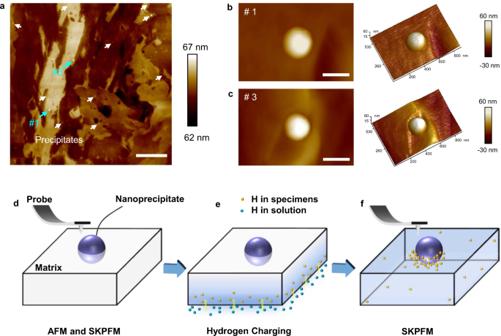Fig. 1: Atom force microscope (AFM) maps of the precipitates in martensite matrix and schematic illustrations of the experiment procedure. aTopography map for martensite matrix including nanoprecipitates.b,c. Tomography maps of precipitate #1 and #3 corresponding to marked by the cyan arrows in panelarespectively.d–f. Schematic illustrations of the scanning Kelvin probe force microscopy (SKPFM) experiment procedure. Scale bars ina4 μm, inb,c200 nm. In situ SKPFM experiment Figure 1a–c show the atom force microscope (AFM) topography map of the high-strength low-alloyed steel sample, featuring with round-shaped nanoprecipitates uniformly dispersed in the martensite matrix (Supplementary Fig. 1 for a bright-field TEM image of the steel microstructure). After an initial SKPFM scan (Fig. 1d ), the plate sample is transferred onto a device for charging hydrogen on the backside for 25 min (Fig. 1e ). The electrochemical charging process is carried out in a 0.2 mol L −1 NaOH and 0.22 g L −1 thiourea electrolyte with a current density of 12 mA cm −2 . During the process, hydrogen atoms form on the backside of the sample and, driven by the concentration gradient, gradually diffuse along the sample thickness direction to the oxide film on the front surface of the plate sample and then desorb after recombination into hydrogen gas or oxidation in the air into water molecules. The trend of hydrogen content evolution within the sample is roughly simulated (Supplementary Fig. 2 and Supplementary Method 1 ) [25] , [26] . Fig. 1: Atom force microscope (AFM) maps of the precipitates in martensite matrix and schematic illustrations of the experiment procedure. a Topography map for martensite matrix including nanoprecipitates. b , c . Tomography maps of precipitate #1 and #3 corresponding to marked by the cyan arrows in panel a respectively. d – f . Schematic illustrations of the scanning Kelvin probe force microscopy (SKPFM) experiment procedure. Scale bars in a 4 μm, in b , c 200 nm. Full size image The sample is immediately transferred back for SKPFM imaging after the hydrogen charging (Fig. 1f ). Referring to the sample preparation process (see Methods), a thin film of oxides exists on the sample surface which should mainly contains iron oxides, hydroxides, and oxyhydroxides; when hydrogen atoms arrive at the oxide film, they would partially reduce these compounds, leading to a decrease in the work function [27] , [28] . As such, by detecting the Volta potential difference (simply referred to as “potential” in the following and see Methods for the definition), the in situ SKPFM can actually monitor the gradual infusion and egression of hydrogen as the electrochemically-charged hydrogen ingress on the front surface [29] , [30] , [31] . Thereby, two types of apparently distinct responses at the precipitate/matrix interface are revealed; representative cases of each type are shown in the time-lapsed SKPFM images in Fig. 2 and described in the following. Note that, since hydrogen atoms would likely recombine to desorb or be oxidized by oxygen in air and desorb as water, their activity in the oxide and hence the detected potential drop are not high [31] . Fig. 2: In situ scanning Kelvin probe force microscopy (SKPFM) measurement on hydrogen-precipitate interactions. a – d Potential maps of precipitate #1 measured at uncharged state and sequential hydrogen-charged states at t = 160 min, 1320 min, 4940 min. e Potential profiles along the yellow dotted line in panels a , d . f – i Potential maps of precipitate #3 measured at uncharged state and sequential hydrogen-charged states at t = 360 min, 1200 min, 4860 min. j Potential profiles along the yellow dotted line in panels f , i . All scale bars, 200 nm. Full size image In situ SKPFM on the hydrogen trapping by the precipitate Note that before hydrogen charging, both precipitates interiors have lower potential than the martensite matrix (Fig. 2a, f ). As hydrogen diffuses toward the front surface, potential of the region gradually decreases and reaches the minimum at ~160 mins (Fig. 2b ). Subsequently, when hydrogen desorption overruns ingression, potential of the region gradually increases (Fig. 2c ). Incidentally, the simulated hydrogen concentration evolution on the sample surface shows a similar trend (Supplementary Fig. 2 ), albeit quantitative correlation between hydrogen concentration and the potential is yet to be explored. Remarkably, when hydrogen desorption almost completes at 4940 mins, potential of the interface is the lowest compared with the precipitate interior and the matrix (Fig. 2d ). Additionally, compared with the pristine state, the potential drops more steeply at the interface than those at the matrix and the precipitate (Fig. 2e ). These phenomena imply that the border area traps more hydrogen than the matrix. Temporal evolution of the measured potential drop also supports this (Supplementary Fig. 3 ). In situ SKPFM on the hydrogen exclusion by the precipitate In stark contrast to the above observation, the area nearby the border of the other precipitate shows totally different response upon hydrogen ingression (Fig. 2f–j ). As hydrogen diffuses toward the front surface, potential of the interface is characteristically higher than those of the matrix and the precipitate interior; this is manifested vividly by the “bright ring” features in the SKPFM images (Fig. 2g, h ). This feature remains even when hydrogen desorption almost completes at 4860 min (Fig. 2i ), suggesting that the area nearby the border of this precipitate is less prone to trap hydrogen than the matrix. Note that the above distinct scenarios of precipitate-hydrogen interaction are repeatedly found in several independent tests with different nanoprecipitates (Supplementary Fig. 4 ). Particularly, 240 hrs after the initial hydrogen charging, the potential of the interface of precipitate #2 is still lower than that of the matrix (Supplementary Fig. 4c ), suggesting that the interface provides a deep trap for hydrogen. Since precipitates with different hydrogen trapping behaviours have been found simultaneously in the same martensite lath (Supplementary Fig. 4e, f ), these distinct behaviours should not be attributed to the matrix. To pinpoint the underlying factor that governs the hydrogen-trapping characteristics of these precipitates, in the following, we compare the phases of the precipitates and atomic-scale structural and chemical features of the interface. Precipitate phase analysis By using the focused ion beam (FIB), the precipitates and surrounding matrix are lifted out and thinned for STEM characterization (Fig. 3a–c ). Note that precipitate #2 with the same hydrogen-trapping characteristic as precipitate #1 is chosen for the analysis (see its SKPFM result in Supplementary Fig. 4c and Supplementary Note 1 ). First of all, as shown by the high-angle annular dark-field scanning transmission electron microscopy (HAADF-STEM) images and energy-dispersive X-ray spectroscopy (EDS), the two precipitates have similar composition of mainly Ti, C, and S (Fig. 3d–i ). Note that the EDS quantification on C content is not accurate due to the carbon contamination that is commonly encountered in STEM imaging. Further, high-resolution transmission electron microscopy (HRTEM), STEM and the selected area electron diffractions (SAED) of the precipitates are acquired (Fig. 4a, b, d, e ). After scrutinizing all reported phases containing Ti-C-S, Ti-C, or Ti-S, it is found that only the Ti 2 CS phase (space group P63/mmc, lattice parameters of a = 0.32 nm and c = 1.13 nm) provides the best match to all the experimental data including the HRTEM image, STEM image, SAED patterns, and EDS quantification results on Ti/S ratio of the precipitates. Fig. 3: Lift-out and scanning transmission electron microscopy energy dispersed X-ray spectroscopy (STEM-EDS) analysis of the precipitates. a–c Identify, lift out, and FIB thinning of the precipitates. d , e STEM images of the precipitates #2 and #3, respectively. f , g EDS mapping of the boxed regions in panels d , e . h , i EDS line data along the yellow line in panels f , g showing the elemental composition across the precipitate/matrix interface. Note that the EDS quantification on C content is not accurate due to the carbon contamination that is commonly encountered in STEM imaging. Scale bars in a 10 μm, in d , e 50 nm, in f , g 20 nm. Full size image Fig. 4: Structure of the precipitate and the precipitate/matrix interface. a–c High-resolution transmission electron microscopy (HRTEM) image of the precipitate #2, electron diffraction pattern of its interface with the matrix, and atomic structure model of the interface constructed based on the mutual orientation, respectively. d – f Scanning transmission electron microscopy (STEM) image of the precipitate #3, electron diffraction pattern of its interface with the matrix, and atomic structure model of the interface constructed based on the mutual orientation, respectively. Note that, in panel e , the precipitate was not oriented exactly on the [100] zone axis but tilted 7.6° away from the zone axis (Supplementary Fig. 5 ); as such, the diffraction spot of the (010) plane is invisible; the diffraction spot of the (001) in panel e is a forbidden reflection visible due to double diffraction. Insets in panels a, d are corresponding projection view of the Ti 2 CS atomic models and simulated HRTEM images. Scale bar in a , d , 1 nm, in b , e 5 nm −1 . Full size image Structures of the precipitate/matrix interfaces Mutual orientations of the precipitate and the surrounding matrix are determined by using the SAED analysis. The [ \(1\bar{2}1\) ] Ti2CS zone axis of precipitate #2 is roughly parallel to the [001] matrix axis of the matrix (Fig. 4b ); the [100] Ti2CS axis of precipitate #3 tilts 7.6° away from the [102] matrix axis of the matrix (Fig. 4e and Supplementary Fig. 5 for more details on determining the mutual orientation). These orientation relation between the precipitate and the martensite matrix is neither the Baker–Nutting orientation relationship [32] nor the Nishiyama-Wassermann (N-W) orientation relationship [33] that are conventionally found in coherent or semi-coherent TiC precipitates. Based on the mutual orientation analysis, atomic models of the interfaces are manually constructed by using an QuantumATK software [34] , which clearly illustrated the incoherent precipitates/matrix interfaces (Fig. 4c, f ). Note that these models are only for illustration purposes and requires atomic-scale characterization in 3 dimensions to be accurate [35] , [36] . Chemical features of the precipitate/matrix interfaces Note that the EDS line-scan data across the interface indicates no significant elemental segregation at the interfaces (Fig. 3h, i ). To explore possible carbon or sulfur vacancies on the interface, we performed electron energy loss spectroscopy (EELS) analysis on the L 2, 3 core-loss edges of Ti for precipitates #2 (Fig. 5a ) and #3 (Fig. 5b ). Comparing the precipitation #2 interior Ti-L 2, 3 peaks (463.1 eV for Ti-L 2 and 457.8 eV for Ti-L 3 ), the interface Ti-L 2, 3 peaks shift 0.2 eV and 0.4 eV, respectively to lower energies. As for the precipitate #3, the interface Ti-L 2, 3 peaks shift 0.3 eV and 0 eV respectively to higher energies, compared with the precipitation interior (463.2 eV for Ti-L 2 and 457.9 eV for Ti-L 3 ). Referring to literatures [37] , shifting of the Ti-L 2, 3 peaks to lower energies corresponds to a decrease of the Ti valence state. Therefore, the above EELS data indicates that Ti on the interface of precipitation #2 and matrix is more reduced than Ti on the interface of precipitation #3 and matrix, likely due to the presence of more C or S vacancies. Fig. 5: Electron energy loss spectroscopy (EELS) analysis on the Ti L 2, 3 core-loss edges of precipitate interior and interface with the martensite matrix. a EELS spectrums of precipitate #2 interior and interface. b EELS spectrums of precipitate #3 interior and interface. Dash lines indicate the L 2 and L 3 peak positions. Full size image To evaluate the effect of C and S vacancies on the hydrogen trapping ability, we performed density function theory (DFT) calculations on the solution energy of H atom at C and S vacancies within the Ti 2 CS precipitate (see Methods for details). As shown in Table 1 , the calculated solution energy of hydrogen at C vacancy and S vacancy are −0.75 eV and −0.38 eV, respectively; while that of α-Fe (tetrahedral site) is markedly higher (0.23 eV). An interesting question arises as how the area nearby the border of precipitate #3 excludes hydrogen even though it may not contain as much C/S vacancies as the interface of precipitate #2 and the matrix. Table 1 The density function theory (DFT) and nudged elastic band (NEB) calculation results. Full size table Strain state on the precipitate/matrix interfaces The strain state of the matrix right next to the interface is analyzed by directly interpreting the atoms-column positions in atomic-resolution HAADF-STEM images. We used the CalAtom [38] software to determine the precise position of each atomic column within the region of without obvious dislocations to avoid the influence of dislocation cores on the strain measurement (Fig. 6a, b and Supplementary Fig. 6 ). Note that the CalAtom software employs a multiple-ellipse fitting algorithm to determine the positions of the atomic columns with high precision, which has been widely applied in literatures [39] , [40] . Following the strain analysis method in the literature [41] , atomic strain maps are generated by comparing the nearest-neighbor distances in two crystallographic directions (namely \(\left[1\bar{1}0\right]\) and [110]) separately to their reference values. For visualization, the strain at each atomic column is color-coded and plotted into a 2D map (Fig. 6c, d ). We measured and compared the strain values of the martensite matrix within 3 nm from the interface (Fig. 6a, b ) and 150 nm afar from the interface (Supplementary Fig. 6a, b ). Separate strain maps are generated for each of \(\left[1\bar{1}0\right]\) and [110] crystallographic directions. All strain values within the area of interest are statistically plotted (Supplementary Fig. 7a ). The statistical measurements suggest that, the lattices nearby the border of precipitate #2 is tensile-strained by, on average, 2.2% along the [110] direction and 1.7% along the \(\left[1\bar{1}0\right]\) direction; as for the precipitate #3, the region right by the border is compressively strained by, on average, −1.3% along the [110] direction and −0.6% along the \(\left[1\bar{1}0\right]\) direction. Fig. 6: Atomic strain maps nearby the border of the precipitates. a , b The filtered atomic resolution high-angle annular dark field scanning transmission electron microscopy (HAADF-STEM) images of the martensite matrix nearby the interfaces. Yellow dash lines mark the region for the atomic strain analysis. Note that, in each case, the reference region is within the same martensite lath and ~150 nm afar from the interface (Supplementary Fig. 6 ). c , d Atomic strain maps of the region within 3 nm distance from the interfaces. e , f Density function theory (DFT) calculations on the solution energy of H atom at the tetrahedral interstitial sites and corresponding tetrahedral volume in α-Fe of precipitate #2 (green dash lines) and precipitate #3 (yellow dash lines). Note that the same magnitude of strains are applied to the [110] and \([1\bar{1}0]\) directions; and the positive and negative values of strain represent tensile and compressive strains, respectively. The [001]+1% notion in the legend means that an additional 1% tensile strain was applied along the [001] direction. Scale bars in panels a , b , 2 nm. Full size image To further evaluate the effects of above strains on the hydrogen trapping, we carried out DFT calculations on the solution energy of H atom at the tetrahedral interstitial site and the tetrahedral volume of α-Fe at the above strained states (see Methods for details). As shown in Table 1 , the solution energy of tensile strained α-Fe is less than that of compressively strained α-Fe, while the tetrahedral volume of the former is larger than the latter, implying that the strain state corresponding to the case of precipitate #2 is more favorable to trap hydrogen than that of the precipitate #3. In other words, the tensile strain fields facilitate the dissolution of H while the compressive strain suppress it. When additional 1% tensile/compressive strain was applied along the [001] direction (i.e., parallel to the observation direction of the TEM experiment) in the DFT calculation, the above finding persists (Fig. 6e, f ). It is well known that the solution of hydrogen will lower the work function of the oxide film on the sample surface [27] , [28] and hence lowering the potential as detected by the SKPFM [42] , [43] , [44] . Note that the surface species on the Ti 2 CS precipitates and the martensite matrix are likely different, and hence their responses to hydrogen may not be the same; therefore, we cannot conclude on the relative H concentration within the precipitate by comparing the potential changes with those on the matrix. However, the changes in potential of precipitate interior decreasing and recovering in the same way by the infusion and egression of hydrogen need consideration. H flux may have entered the Ti 2 CS precipitates and contributed to the measured potential drop at the precipitate surface during the in situ SKPFM experiments. In principle, H atoms entering the precipitates will not affect the trapping and diffusion of H on the interfaces. (Supplementary Discussion 1 for more on this point). Nevertheless, the oxide film in the vicinity of the interface is reasonably the same as that on the matrix afar (Supplementary Discussion 2 and Supplementary Fig. 8 ); and hence their responses to H should be the same. The SKPFM results of precipitate #1 showing the lowest potential and largest potential drop at the interface (Fig. 2a–e and Supplementary Fig. 3a, b ) indicate that hydrogen prefers to lodge in the vicinity of the incoherent interface than within the martensite matrix. Whereas the SKPFM results of precipitate #3, showing higher potential at the interface than within the martensite matrix (Fig. 2f–j and Supplementary Fig. 3c, d ), suggest that the interface tend to exclude hydrogen compared with the martensite matrix. More discussions on how we interpreted the SKPFM results can be found in Supplementary Discussion 3 . As corroborated by the repeated results on other precipitates (Supplementary Fig. 4 ), the incoherent interfaces are apparently not reacting in the same way upon the infusion of hydrogen. This finding can satisfactorily explain the seemingly controversial discoveries in macro- and micro-scale experiments. As for bulk materials wherein a large number of incoherent precipitates coexist, the ensemble-averaged hydrogen trapping ability of the precipitates could be trivial as reflected in many TDS results [20] , [21] . However, when probing individual precipitates, it is fairly possible to capture hydrogen-trapping by incoherent interfaces [23] . Hydrogen-trapping ability of precipitates are conventionally attributed to atomic-scale features of the interface including chemical features such as carbon vacancies [45] and structural features such as misfit dislocations [5] , [14] , [15] , [16] and strains [46] . Though reasonably demonstrated in (semi)coherent precipitates, this is implied more often than proven in incoherent precipitates. The diverse hydrogen trapping behaviours may root in the fact that the incoherent interfaces easily vary with precipitate-matrix mutual orientations and the precipitate formation conditions [15] , [47] . Therefore, pin-pointing the mechanism of hydrogen trapping by the incoherent interfaces indispensably requires characterizations of the atomic-scale structure and hydrogen trapping behaviours with the same single precipitate, as uniquely enabled here through the in situ SKPFM-FIB-TEM workflow. On chemical features of the interface, the quantitative EDS line-scan results in Fig. 3h, i indicate no obvious elemental segregation on the both interfaces. However, the EELS data shows a minor shift in the Ti L 2, 3 peaks positions, indicating that the valence state of Ti on the surface of precipitate #2 is lower than that of precipitate #3 [37] . This implies that the C and/or S vacancies exist on the surface of precipitate #2. In fact, carbon vacancies are commonly found in alloy carbide precipitates in ferritic steels as have been demonstrated in previous APT results showing the atomic ratios of C and transition metal of the precipitates being lower than the ideal stoichiometry [45] ; in addition, the formation energy of carbon vacancies decreases with the loss of coherency at the TiC/α-Fe interface [46] . The underlying reason for the different contents of surface C/S vacancies may be associated with the formation temperature of the precipitates. Thermal dynamic calculations have proven that concentration of carbon vacancies in alloy carbide precipitates increases with temperature [48] . Given that the incoherent Ti 2 CS precipitates can be formed in a wide temperature window (Supplementary Fig. 9 ), the C/S vacancies are deemed to present with varying concentrations in different precipitates. Additionally, concentration fluctuation of Ti, C, and/or S at the precipitate formation site can also incur the non-stoichiometry at the interface. 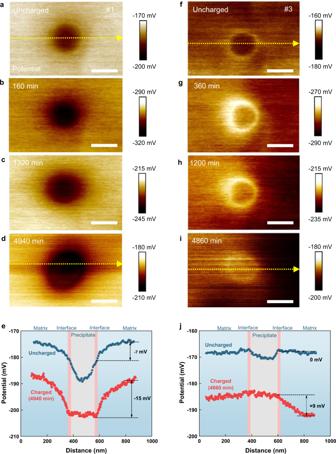Fig. 2: In situ scanning Kelvin probe force microscopy (SKPFM) measurement on hydrogen-precipitate interactions. a–dPotential maps of precipitate #1 measured at uncharged state and sequential hydrogen-charged states att= 160 min, 1320 min, 4940 min.ePotential profiles along the yellow dotted line in panelsa,d.f–iPotential maps of precipitate #3 measured at uncharged state and sequential hydrogen-charged states att= 360 min, 1200 min, 4860 min.jPotential profiles along the yellow dotted line in panelsf,i. All scale bars, 200 nm. Due to the existing difficulty in reasonably constructing the intrinsically non-periodical structure of the incoherent interface, we cannot calculate the solution energies of C/S vacancies on the precipitate surface. Though, our previous studies on coherent interfaces between α-Fe and other precipitates (VC, TiN, NbC) suggest that the solution energies of non-metallic element vacancies on the interface are considerably lower than those inside the bulk precipitate [17] . Moreover, extensive theoretical works suggest that carbon vacancies on the surface of alloy carbide precipitates are deep hydrogen traps [17] , [45] , [49] , and reducing the amount of surface carbon vacancies may lower their hydrogen trapping energy [45] . As such, the C and/or S vacancies on the surface of precipitate #2 are deemed to impart a better hydrogen trapping capability than the surface of precipitate #3. Moreover, the C and S vacancies on the precipitate surface are readily accessible to hydrogen [45] , [46] . On the atomic structure feature of the interface, firstly, mutual orientation analysis shows that interfaces of both precipitates are incoherent in nature (Fig. 4 ). Due to the lack of effective experimental or computational approaches, it is hard to solidly unravel the atomic structures of the interfaces. Nevertheless, as illustrated in Fig. 4c, f , the two interfaces should have different structures with different interstitial sites for anchoring hydrogen. Secondly, strain analysis indicates that the martensite matrix nearby the precipitate #2 are tensile strained while that in the vicinity of precipitate #3 are compressively strained (Fig. 6 ). As corroborated by the DFT calculations, the tensile strain field prompts hydrogen trapping while the compressive strain field nearby precipitate #3 suppresses hydrogen trapping, which are consistent with the SKPFM findings and indicates that tensile strain field is a hydrogen trapping mechanism at the vicinity of incoherent interfaces. Though, the DFT calculations and previous reports [46] suggest that the strain fields are weak hydrogen traps than the C/S vacancies (Table 1 ). The different strain fields surrounding different precipitates may be associated with the atomic structures between the Ti 2 CS precipitates and the martensite matrix. Moreover, the hydrogen-excluding behaviours as shown on the border of precipitate #3 may be associated with the fact that the compressive strains in the nearby matrix increase the solution energy of H. Due to the limitation of the SKPFM resolution, we only probed precipitates of 100 nm or larger in diameter, which are usually formed in the smelting and hot-rolling process in the high temperature range. Though, the findings on the atomistic origins of hydrogen-trapping/exclusion at the precipitates interface are directly applicable to much smaller precipitates with semi-coherent or coherent interfaces wherein non-stoichiometry and elastic strains are common [20] , [45] , thusly paving way for achieving desirable precipitate-hydrogen interaction in steels and coupling of precipitation-strengthening and hydrogen-insensitive designs. For instance, to trap hydrogen from concentrating at vulnerable locations and hence mitigate hydrogen embrittlement, precipitates in steels could be designed with non-stoichiometry and/or desirable strain fields in the surrounding matrix. In fact, this may have been realized in literatures reporting the positive roles of elastic-strain field [17] , [20] , interfacial dislocations [47] , and vacancies [45] around the coherent or semi-coherent precipitates in lowering the hydrogen embrittlement sensitivity of steels. With the advancement of SKPFM resolution [44] , the experimental methods as demonstrated here may enable direct investigation on much smaller precipitates. Above all, the dynamic interactions between hydrogen and incoherent precipitates are captured. Atomic-scale structural and chemical features of the very interfaces suggest that carbon/sulfur vacancies on the precipitate surface and strain of the matrix nearby the interface determine the hydrogen-trapping characteristics of the incoherent interfaces. The findings unravel the perplexing hydrogen trapping behaviours of incoherent precipitates. Since direct imaging of solute hydrogen atoms is difficult [50] , our study demonstrates a viable method to directly probe the hydrogen trapping behavior and the structural/chemical characteristics of exactly the same site, paving way for the study on the atomic origin of hydrogen-assisted cracking, especially when structures of the associated defects (such as grain boundaries and matrix/inclusion interfaces) are intrinsically diverse. Materials A high-strength low-alloy martensitic steel was used for this study. Composition of the steel is shown in Supplementary Table 1 . The steel was hot-rolled to 12.7 mm and then cold-rolled to 10 mm. The plate was solution treated at 900 °C for 30 min, quenched in water, tempered at 500 °C for 60 min and then cooled in air. A bright-field TEM image of the martensitic steel is shown in Supplementary Fig. 1 . The hydrogen diffusion coefficient of the steel is measured to be 3.3 × 10 −8 cm 2 s −1 . In-situ SKPFM experiment procedure The steel was cut into plates of 0.49 mm in thickness; the plate specimen was mechanically polished with SiO 2 suspension and then etched with Argon ion for 30 mins to remove the native oxide and contaminations on the surface. Thereafter, when the fresh surface was exposed to air, it should have been oxidized again by the oxygen in air, forming a very thin oxide film on the sample surface. The SKPFM experiments were conducted in the tapping mode using a dimension Nanoscope V (Veeco Instruments Inc.). The Volta potential difference (simply referred to as potential in the main text) was obtained in situ before and after hydrogen charging, and is defined by ( φ sample – φ tip )/ e , where φ sample and φ tip are the work function of sample and tip, respectively, and e represents the value of the elementary charge [43] , [51] . In SKPFM, φ tip is a constant; therefore, the potential is proportional to φ sample which changes with the local hydrogen concentration [31] . The cantilever used in our study has a spring constant of 2.8 N m −1 , a resonant frequency of 60–100 kHz, and a standard PtIr-coated silicon tip with a <25 nm curvature. Lift height was set to 60 nm. The SKPFM experiments were carried out in air at room temperature and relative humidity of 38 ± 1%. The system was calibrated by using a high-quality highly-oriented pyrolytic graphite (HOPG) [52] prior to the experiment to ensure the accuracy of the potential measurements. TEM sample preparation and characterization The TEM sample was prepared by using a Thermo Fisher Helios dual-beam system. To protect the precipitate from damage, carbon, and platinum layers were deposited with the electron beam on top of the precipitate before the FIB milling. TEM, STEM, and EDS analysis were performed on a Thermo Fisher ThemisZ TEM equipped with both probe and imaging lens spherical aberration correctors. EELS was acquired with a Gatan GIF Continuum 1065 instrument. Density Function Theory calculations The DFT calculations were performed in the Vienna ab initio Simulation Package (VASP) [53] . Hydrogen diffusion energy barrier were mapped by the minimum energy reaction path with the nudged elastic band (NEB) [54] method. The core electrons were modeled with the projector-augmented-wave (PAW) method [55] . The exchange and correlation functional of Perdew-Burke-Ernzerhof (PBE) was adopted within the framework of generalized gradient approximation (GGA) [56] . An energy cut-off of 400 eV and 5 × 5 × 5, 3 × 3 × 3 k-point meshes were used to ensure calculation accuracy for α-Fe and Ti 2 CS, respectively. All of the calculations were carried out as spin-polarized and the forces on all the atoms were less than 0.02 eV Å −1 during the geometrical optimizations. 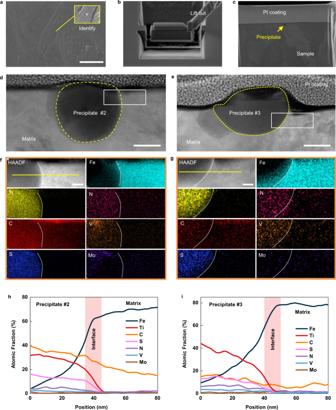Fig. 3: Lift-out and scanning transmission electron microscopy energy dispersed X-ray spectroscopy (STEM-EDS) analysis of the precipitates. a–cIdentify, lift out, and FIB thinning of the precipitates.d,eSTEM images of the precipitates #2 and #3, respectively.f,gEDS mapping of the boxed regions in panelsd,e.h,iEDS line data along the yellow line in panelsf,gshowing the elemental composition across the precipitate/matrix interface. Note that the EDS quantification on C content is not accurate due to the carbon contamination that is commonly encountered in STEM imaging. Scale bars ina10 μm, ind,e50 nm, inf,g20 nm. 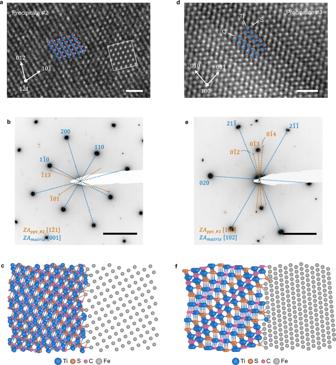Fig. 4: Structure of the precipitate and the precipitate/matrix interface. a–cHigh-resolution transmission electron microscopy (HRTEM) image of the precipitate #2, electron diffraction pattern of its interface with the matrix, and atomic structure model of the interface constructed based on the mutual orientation, respectively.d–fScanning transmission electron microscopy (STEM) image of the precipitate #3, electron diffraction pattern of its interface with the matrix, and atomic structure model of the interface constructed based on the mutual orientation, respectively. Note that, in panele, the precipitate was not oriented exactly on the [100] zone axis but tilted 7.6° away from the zone axis (Supplementary Fig.5); as such, the diffraction spot of the (010) plane is invisible; the diffraction spot of the (001) in paneleis a forbidden reflection visible due to double diffraction. Insets in panelsa, dare corresponding projection view of the Ti2CS atomic models and simulated HRTEM images. Scale bar ina,d, 1 nm, inb,e5 nm−1. 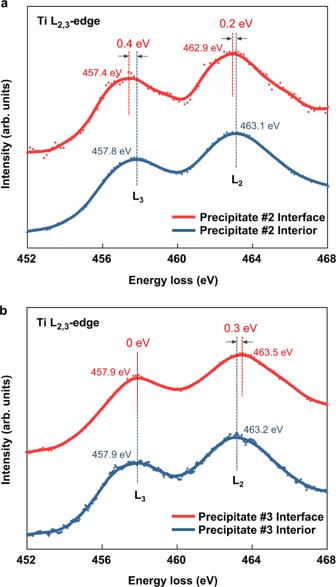Fig. 5: Electron energy loss spectroscopy (EELS) analysis on the Ti L2, 3core-loss edges of precipitate interior and interface with the martensite matrix. aEELS spectrums of precipitate #2 interior and interface.bEELS spectrums of precipitate #3 interior and interface. Dash lines indicate the L2and L3peak positions. 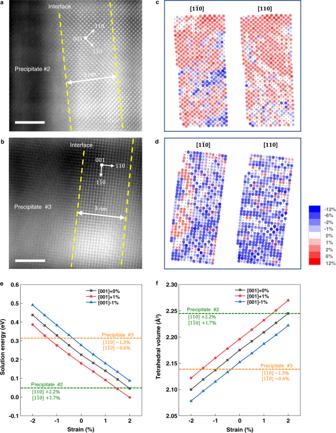Fig. 6: Atomic strain maps nearby the border of the precipitates. a,bThe filtered atomic resolution high-angle annular dark field scanning transmission electron microscopy (HAADF-STEM) images of the martensite matrix nearby the interfaces. Yellow dash lines mark the region for the atomic strain analysis. Note that, in each case, the reference region is within the same martensite lath and ~150 nm afar from the interface (Supplementary Fig.6).c,dAtomic strain maps of the region within 3 nm distance from the interfaces.e,fDensity function theory (DFT) calculations on the solution energy of H atom at the tetrahedral interstitial sites and corresponding tetrahedral volume in α-Fe of precipitate #2 (green dash lines) and precipitate #3 (yellow dash lines). Note that the same magnitude of strains are applied to the [110] and\([1\bar{1}0]\)directions; and the positive and negative values of strain represent tensile and compressive strains, respectively. The [001]+1% notion in the legend means that an additional 1% tensile strain was applied along the [001] direction. Scale bars in panelsa,b, 2 nm. During the transition state calculation, the atoms were allowed to fully relaxed until the forces on all atoms were less than 0.05 eV Å −1 . The total energy was converged to 10 −5 eV for the Self-Consistent Field (SCF) calculation. The solution energy of an H atom at the trapping sites (tetrahedral interstitial site of α-Fe, C vacancy and S vacancy in Ti 2 CS precipitate) is defined by, 
    E_sol=E_trap+H-E_trap-1/2E_H_2
 (1) where E trap+H is the total energy of the unit-cell that dissolves one H atom, E trap is the total energy of the same unit-cell without H, and \({E}_{{{{{{{\rm{H}}}}}}}_{2}}\) is the energy of an isolated hydrogen molecule. The atomic structures used in the above calculation were shown in Supplementary Fig. 10 .